Enhanced thermal transport at covalently functionalized carbon nanotube array interfaces It has been more than a decade since the experimental demonstration that the thermal conductivity of carbon nanotubes can exceed that of diamond, which has the highest thermal conductivity among naturally occurring materials. In spite of tremendous promise as a thermal material, results have been disappointing for practical thermal systems and applications based on nanotubes. The main culprit for the dramatic shortfall in the performance of nanotubes in practical systems is high thermal interface resistance between them and other components because of weak adhesion at the interface. Here we report a sixfold reduction in the thermal interface resistance between metal surfaces and vertically aligned multiwall carbon nanotube arrays by bridging the interface with short, covalently bonded organic molecules. These results are also significant for single and multilayer graphene applications, since graphene faces similar limitations in practical systems. Thermal transport limits the performance of many technologies such as micro and nano electronics and optoelectronics, micro–electro–mechanical systems, and important energy technologies including thermoelectric generation, concentrated photovoltaic systems and electrochemical batteries [1] , [2] , [3] , [4] , [5] . Although significant advances such as microchannels, heat pipes and thermoelectrics [6] , [7] have been made in thermal devices for various applications in the last few decades, performance is often limited by the interface between these devices and the components whose temperature needs to be controlled [7] . For example, modern microprocessors are limited by a thermal bottleneck—the need to get the heat out of the chips. Efficient heat transfer is also a major issue for concentrated photovoltaic systems since difficulty in removing waste heat reduces the efficiency of the solar cell. In spite of significant advances in nanostructured high-figure-of-merit thermoelectric materials, the results in integrated systems have been suboptimal because of poor thermal transport across interfaces as demonstrated by one of the co-authors [7] . Nanostructured carbon-based materials (graphene and nanotubes) have exceptionally high thermal conductivities [8] , [9] ; however, their use for thermal management has been limited due to high thermal interface resistances in nanostructured systems [10] , [11] , [12] . Interfaces between dissimilar materials often control thermal transport, especially at the nanoscale, where the importance of interfaces relative to bulk material properties is substantially increased [13] . Thermal interface resistance arises from differences in the intrinsic properties of the contacting materials (acoustic impedance, phonon density of states) [14] , contact geometry (real versus apparent contact area) and the strength of atomic-scale interactions at the interface. For carbon nanotube (CNT) array-based systems, the interface resistance to the substrate on which the CNT arrays are grown can be significantly lower depending on the growth conditions than the other mating surface. The main reason is the difference in adhesion. On the growth side CNTs are covalently bonded to the catalyst particles, while contacts with the opposite surface occur through weak van der Waals interactions resulting in poor adhesion. One of the co-authors [15] and others [16] have shown that weak adhesion leads to significant increase in the interface resistance. In this work we have increased adhesion between CNT arrays and either noble or reactive metal contacts by bridging the interface with short, covalently bonded organic molecules. The significantly increased adhesion, now exceeding that to the growth substrate, led to a dramatic, approximately sixfold reduction in the thermal interface resistance of the CNT array contact. Aminopropyl-trialkoxy-silane (APS) reduced the CNT array–aluminium interface resistance to 0.6±0.2 mm 2 K W −1 , while cysteamine reduced the CNT array–gold resistance to 0.8±0.2 mm 2 K W −1 . Functionalized CNT thermal interfaces were shown to be stable in air for many months and resistant to thermal stress was up to 180 °C. We were also able to independently determine the intrinsic CNT interface resistance and the fraction of the CNT array contributing to thermal transport. Since our technique avoids destructive solution-phase processing, this development may lead to the practical integration of CNT arrays for thermal management in microelectronic devices [17] . Functionalization schemes for CNT–metal interfaces Our experimental approach to enhance thermal transport at CNT–metal interfaces is outlined in Fig. 1 . We grew vertically aligned CNT arrays on Si wafers using chemical vapor deposition (CVD) and evaporated thin Al or Au films on glass microscope cover slips. The CNT arrays were exposed to an air plasma, which removed the amorphous carbon layers usually present at the surface of chemical vapor deposition (CVD)-grown arrays, and oxidized the ends of the CNTs. The metal films were amine-functionalized using one of two different reaction schemes, as shown in Fig. 2 . Al films were functionalized with a silane-based chemistry suitable for reactive oxide-forming surfaces including Si and Ti (Al-APS-CNT), while Au was functionalized with a cysteamine-based chemistry suitable for noble metals forming thiol bonds including Cu and Ag (Au-Cyst-CNT). The oxidized CNT arrays were then bonded to the amine-functionalized metal surfaces by allowing the metal amine groups to react with the CNT carboxylate groups. This approach involved only dry processing of the CNT arrays, avoiding capillary collapse from surface tension effects during wet chemical processing [18] . Two types of control samples were also prepared from the same growth wafer, with either as-grown or plasma-oxidized CNTs bonded to plasma-cleaned but non-functionalized Al or Au surfaces. 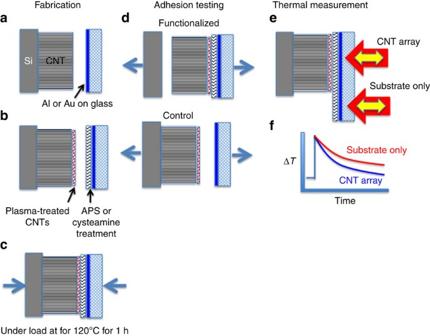Figure 1: Scheme to enhance and characterize thermal transport at CNT–metal interfaces. (a) Vertically aligned CNT arrays were grown on silicon, and Al or Au films were deposited on glass. (b) CNT arrays were exposed to oxygen plasma, while the metal films were amine-functionalized using aminopropyl-trialkoxysilane [Al] or cysteamine [Au]. (c) CNT arrays were covalently bonded to the functionalized metal films by heating under compressive loads. Identical CNT arrays were bonded to plasma-cleaned but non-functionalized metal films as controls. (d) Covalently functionalized samples failed at the CNT–growth substrate interface during adhesion testing, while non-functionalized samples (controls) failed at the CNT–metal interface at much lower loads. (e) Thermal transport measurements were made by heating the metal films with ultrafast laser pulses and then monitoring cooling by thermoreflectance. (f) Differential measurements compared the relative cooling rates between regions of the metal film contacting the CNT arrays (blue) and regions contacting only the glass substrate (red). Figure 1: Scheme to enhance and characterize thermal transport at CNT–metal interfaces. ( a ) Vertically aligned CNT arrays were grown on silicon, and Al or Au films were deposited on glass. ( b ) CNT arrays were exposed to oxygen plasma, while the metal films were amine-functionalized using aminopropyl-trialkoxysilane [Al] or cysteamine [Au]. ( c ) CNT arrays were covalently bonded to the functionalized metal films by heating under compressive loads. Identical CNT arrays were bonded to plasma-cleaned but non-functionalized metal films as controls. ( d ) Covalently functionalized samples failed at the CNT–growth substrate interface during adhesion testing, while non-functionalized samples (controls) failed at the CNT–metal interface at much lower loads. ( e ) Thermal transport measurements were made by heating the metal films with ultrafast laser pulses and then monitoring cooling by thermoreflectance. ( f ) Differential measurements compared the relative cooling rates between regions of the metal film contacting the CNT arrays (blue) and regions contacting only the glass substrate (red). 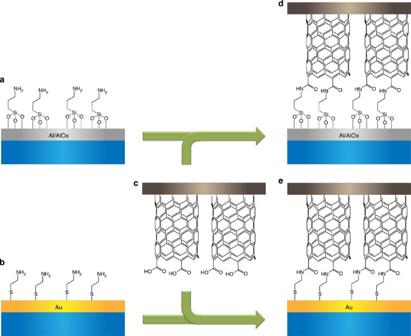Figure 2: Chemical functionalization schemes. (a) Al was cleaned by oxygen plasma and then dipped in an aminopropyl triethoxysilane–ethanol solution, forming metal-O-Si-O bonds to short hydrocarbon chains terminated by amine groups. This reaction also works on Si substrates. (b) Au was cleaned by oxygen plasma and then dipped in a cysteamine–toluene solution forming Au-S bonds to short hydrocarbon chains terminated by amine groups. (c) CNT arrays were plasma-treated to generate carboxylate, hydroxyl and other polar groups. Metal surfaces passivated with amine groups reacted with CNT carboxylate groups forming covalent bonds by elimination of H2O for both (d) Al-APS-CNT and (e) Au-Cyst-CNT samples. Full size image Figure 2: Chemical functionalization schemes. ( a ) Al was cleaned by oxygen plasma and then dipped in an aminopropyl triethoxysilane–ethanol solution, forming metal-O-Si-O bonds to short hydrocarbon chains terminated by amine groups. This reaction also works on Si substrates. ( b ) Au was cleaned by oxygen plasma and then dipped in a cysteamine–toluene solution forming Au-S bonds to short hydrocarbon chains terminated by amine groups. ( c ) CNT arrays were plasma-treated to generate carboxylate, hydroxyl and other polar groups. Metal surfaces passivated with amine groups reacted with CNT carboxylate groups forming covalent bonds by elimination of H 2 O for both ( d ) Al-APS-CNT and ( e ) Au-Cyst-CNT samples. Full size image Mechanical characterization Enhanced CNT–metal adhesion was confirmed by mechanical testing. Tensile load was applied between the Si-CNT growth substrate and the bonded surface while monitoring strain. The control samples either failed spontaneously under their own weight (<0.1 kPa) or under low tensile stress (<8 kPa) at the CNT–metal interface, while functionalized samples failed at the Si-CNT growth interface under significantly larger stress (40–70 kPa), resulting in complete transfer of the vertically aligned CNT arrays from the growth substrate to the amine-functionalized metal. While the CNTs bond strongly to their growth catalysts, the catalyst–growth substrate adhesion is highly dependent on substrate preparation and catalyst deposition method. In many cases, CNT arrays can be removed intact from growth substrates [19] . As our growth substrate interface failed first, our adhesion tests give only a lower limit on CNT array-functionalized interface adhesion. Thermal transport measurements We characterized the CNT–metal thermal interface resistance by heating the metal films with laser pulses passing through the glass cover slips, and then monitoring the subsequent cooling process through temperature-dependent changes in the optical reflectivity as heat flowed from the metal into both the glass substrate and the CNT array. Differential measurements compared the relative cooling rates for regions of the metal in contact with CNT arrays and regions supported only by the glass substrate, as shown schematically in Fig. 1f . Characteristic cooling times are a few nanoseconds, too fast to measure in real time, so we used the time-domain thermoreflectance (TDTR) optical pump-probe technique [20] . The experimental configuration was suggested by the liquid–solid TDTR studies of Schmidt et al. [21] The effective CNT array thermal-interface resistance depends on the intrinsic thermal interface conductance G for metal–CNT contacts and also on the fraction of individual CNTs that make good thermal contacts and contribute to transport. As there are some variations in the length and orientation of the CNTs in the array, only a minority can be expected to contribute. Here we scale the CNT array properties relative to the mass density of HOPG (highly oriented pyrolitic graphite). CVD-grown vertically aligned CNT arrays have about 10% HOPG density [22] and we use this as our reference value. The axial thermal conductivity of multiwall carbon nanotubes (MWCNTs) at room temperature is similar to the in-plane thermal conductivity of graphite, about 2,000 W m −1 K −1 (ref. 8 ). If one CNT in four makes contact, the relative contact density σ contact will be 25%, and the effective area-averaged CNT thermal conductivity will be ~50 W m −1 K −1 . CNT heat capacity also scales with σ contact while interface resistance is the inverse of σ contact G . The characteristic length scale for thermal transport across interfaces is defined by L int = Λ / G , where Λ is the bulk thermal conductivity. G controls transport over distances smaller than L int . For an experiment to be sensitive to changes in G , thermal transport should ideally be measured at this length scale. This can be achieved through experiments in the time domain. When a surface is periodically heated, exponentially decaying thermal waves propagate away from the surface with a decay length , where f is frequency and c v is the volumetric specific heat. At 1 MHz, L harmonic is ~20 μm for CNTs, 5 μm for Si and 0.5 μm for glass. We investigated the effect of functionalization on CNT array–metal interface thermal transport using the TDTR at the relevant length scales. Multifrequency TDTR measurements were critical in determining, independently, both G and σ contact for the CNT interface. The lock-in phase-shift as a function of pump–probe delay is the experimental observable in TDTR measurements. TDTR phase shifts at 9 MHz pump modulation and associated fits are shown in Fig. 3 for Al-APS-CNT and Au-Cyst-CNT samples. The data can be fit by a range of different ( G , σ contact ) combinations as shown in Fig. 3d . The results could either be explained by a relatively small fraction of CNTs in contact with a relatively high intrinsic interface conductance—for example, σ contact =4% CNT with G=500 MW m −2 K −1 —or by a larger σ contact with a smaller G —for example, 70% CNT and 20 M m −2 K −1 . 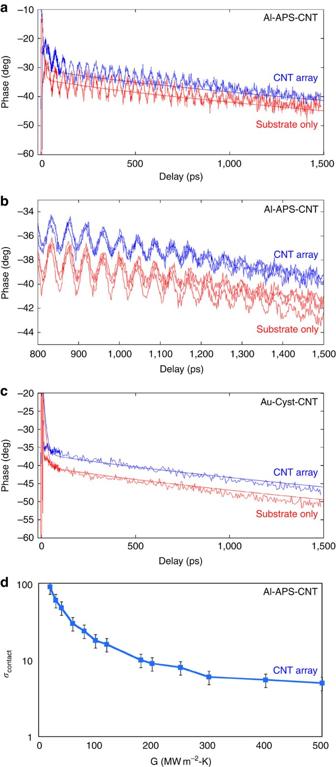Figure 3: Experimental thermal data with model fits. Raw TDTR experimental data along with model fits from one location (a) and from various locations (b) of an Al-APS-CNT sample, and from an Au-Cyst-CNT sample. (c) The CNT contact produces a positive phase shift approximately independent of pump-delay. The oscillations visible in the Al data result from optical probe–pulse reflections from the thermal shock wave propagating in the glass. This effect is much weaker for Au. (d) Locus of (G,σcontact) combinations that produce an acceptable fit to the 9-MHz Al-APS-CNT data. Figure 3: Experimental thermal data with model fits. Raw TDTR experimental data along with model fits from one location ( a ) and from various locations ( b ) of an Al-APS-CNT sample, and from an Au-Cyst-CNT sample. ( c ) The CNT contact produces a positive phase shift approximately independent of pump-delay. The oscillations visible in the Al data result from optical probe–pulse reflections from the thermal shock wave propagating in the glass. This effect is much weaker for Au. ( d ) Locus of ( G , σ contact ) combinations that produce an acceptable fit to the 9-MHz Al-APS-CNT data. Full size image To determine G and σ contact independently, we made additional TDTR measurements at modulation frequencies of 0.8 and 2.3 MHz. Reducing the pump modulation frequency increases the penetration depth of thermal waves and changes the relative influence of G and σ contact . Experimental results for the three frequencies are shown in Fig. 4 . The differential phase shifts for functionalized CNT array contacts were approximately six times greater than for dry (unfunctionalized) contacts, showing a strong enhancement in thermal transport because of covalent interface functionalization. We also see that the differential phase shift is only weakly dependent on modulation frequency. To analyse these results we simulated phase shifts for poor (30 MW m −2 K −1 ) to very good (360 MW m −2 K −1 ) interface conductance G as a function of σ contact at both 9 and 1 MHz ( Fig. 5 ) for a 77 nm Al/Ti film on glass with a 175 MW m −2 K −1 metal–glass interface resistance and a 16 μm pump spot size. The model data showed that when the interface is relatively poor, the differential phase shift increases significantly at lower frequency, while if the interface is relatively good, there will be little change in phase shift as shown in Fig. 5a . In addition, the differential phase shifts increase monotonically with σ contact for all values of G . Figure 5b shows the simulated phase shifts at 9 and 1 MHz for σ contact =5%. 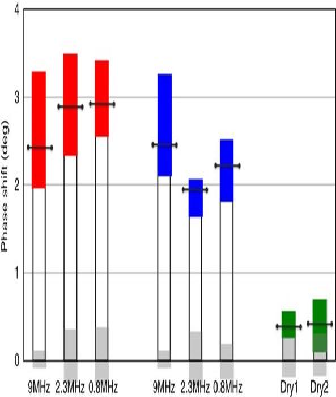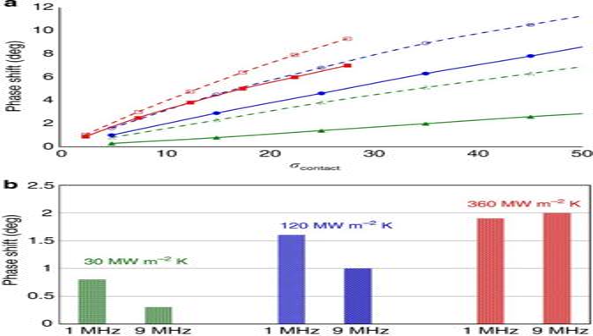Figure 5: Relation between phase shift and (G,σcontact). (a) Simulated phase shifts as a function ofσcontactat 9 MHz (solid lines, filled symbols) and 1 MHz (dashed lines, open symbols) forGvalues of 30 (green triangles), 120 (blue circles) and 360 (red squares) MW m−2K−1. (b) Simulated phase shift calculated for an Al-CNT sample with 5%σcontactat 1 and 9 MHz with poor, good or very good interface conductance. Figure 4: Experimental phase-shift data at multiple frequencies. Observed TDTR differential phase shifts at 0.8, 2.3 and 9 MHz for Al-APS-CNT, Au-Cyst-CNT and two groups of non-functionalized Al-CNT samples (9 MHz only). The extent of the coloured region shows the variation between measurements at different points on the samples. The horizontal lines show the average values. The shaded region at the base of each bar shows the variation between measurements at different reference points outside the CNT contact region. Figure 4: Experimental phase-shift data at multiple frequencies. Observed TDTR differential phase shifts at 0.8, 2.3 and 9 MHz for Al-APS-CNT, Au-Cyst-CNT and two groups of non-functionalized Al-CNT samples (9 MHz only). The extent of the coloured region shows the variation between measurements at different points on the samples. The horizontal lines show the average values. The shaded region at the base of each bar shows the variation between measurements at different reference points outside the CNT contact region. Full size image Figure 5: Relation between phase shift and ( G , σ contact ). ( a ) Simulated phase shifts as a function of σ contact at 9 MHz (solid lines, filled symbols) and 1 MHz (dashed lines, open symbols) for G values of 30 (green triangles), 120 (blue circles) and 360 (red squares) MW m −2 K −1 . ( b ) Simulated phase shift calculated for an Al-CNT sample with 5% σ contact at 1 and 9 MHz with poor, good or very good interface conductance. Full size image The best model fit for the multifrequency TDTR data for Al-APS-CNT gives an intrinsic interface conductance G of 300–500 MW m −2 K −1 with σ contact of 4–5%. The effective interface resistance for the functionalized Al–CNT interface , even with only a few percent of the CNT contributing to thermal transport, was 0.6±0.2 mm 2 KW −1 , the best value reported to date for a vertically aligned CNT array. Similar results were obtained for the Au-Cyst-CNT contacts, where the multifrequency TDTR data gave best fits for G of 250–450 MWm −2 K −1 with σ contact of 4–5%, resulting in R eff =0.8±0.2 mm 2 K W −1 . Assuming the same σ contact for our non-functionalized control samples, G dry was ~50–80 W m −2 K −1 for R eff =3.5±0.5 mm 2 K W −1 . For comparison, thermal resistance ranges from 5 to 10 mm 2 KW −1 for the complete thermal interface in state-of-the-art semiconductor devices [23] . Our mid-range value for effective Al–CNT functionalized interface conductance, 400 MW m −2 K −1 (~ 0.4 nW nm −2 K −1 ) and our typical MWCNT dimensions (18 nm in diameter with 5 nm walls for a cross-section of 204 nm 2 ) correspond to a connected tube interface conductance of 82 nW K −1 , compared with ~14 nW K −1 for dry contacts. The MWCNT length L harmonic probed over our TDTR frequency range is 6.1–20 μm, corresponding to a conductance of 59–18 nW K −1 . Since these contributions have similar magnitudes, we can do a good job of resolving changes in interface resistance. In steady-state heat flow, this gives L int of 5 μm for the CNT interface. Interface conductance will be relatively unimportant for heat flow over distances larger compared with L int . The thermal model used to fit the TDTR data is an idealized model of the physical system. In reality, there will be a distribution of CNT-interface conductance values depending on individual CNT dimensions, contact geometry and number of covalent bonds, while other CNTs will not touch the interface at all. Our model describes this system by separating the CNT population into two groups: a connected fraction, all with the same conductance, and a disconnected fraction that does not participate in thermal transport, similar to the approach of Panzer et al. [24] , [25] The real system will also have tube–tube thermal contacts of ~0.46 nW K −1 (see Supplementary Note 1 ), stabilized by van der Waals interactions, within the vertically aligned MWCNT array. At sufficiently large distances from the interface, these tube–tube contacts will distribute the heat flow uniformly across all the CNTs in the array. One can define a ‘thermal healing length’ [26] L healing where the total conductance of all tube–tube contacts within L healing equals the conductance of an individual CNT of the same length. Thermal transport over distances much greater than L healing will involve the complete CNT array. Transport over distances short compared to L healing will not be significantly influenced by tube–tube contacts. Analysis of our experimental sample shows that L healing is ~30 μm, which is much larger than L harominc , the distance probed in our TDTR experiments; therefore, the data extraction and our conclusions are not affected by CNT–CNT contacts. Finally, the clear difference in the experimental results between the functionalized sample and the non-functionalized control underlines the importance of CNT–metal thermal interface resistance, since heat transport in both sample and control is affected equally by tube–tube thermal contacts. We also explored the effects of contact pressure, aging and thermal stress on CNT thermal interface resistance. Xu et al. [27] reported load-dependent thermal transport for CNT array contacts, although this effect was reduced for their best interfaces. We found no effect of contact pressure for either functionalized or control samples up to 180 kPa, limited by the breaking point of the glass substrates. TDTR measurements conducted on freshly bonded CNT-APS-Al samples and the same samples aged up to 10 months under ambient conditions showed no statistically significant changes, indicating the stability of our interface functionalization. CNT-Cysteamine-Au samples were thermally stressed by annealing for 1 h in an inert atmosphere. No change was observed up to 180 C; however, thermal transport started to decay after 200 C annealing. Understanding the detailed nature of CNT array thermal interface resistance requires measurements made on the appropriate length and timescales. Many groups have conducted steady-state or low-frequency (≤30 kHz) transport [27] , [28] , [29] or ‘3- ω ’ [30] , [31] studies on system incorporating CNT arrays. In a thick system where the CNT heat capacity is only a small fraction of the total heat capacity, the overall thermal resistance of the CNT array can be determined provided it is a thermal ‘bottleneck’, but it is difficult to resolve the individual CNT array properties (density, conductivity, G and σ contact ). Hu et al. [32] imaged a CNT array with an infrared microscope and confirmed that the interface does indeed dominate thermal resistance. Later Panzer et al. [24] , [25] carried out fast real-time measurements (~10 ns time resolution) of the cooling of metal films supported by single-wall CNT arrays using thermoreflectance. They clearly showed that only a small fraction of CNTs (~5–15% of the array,<1% HOPG heat capacity) contributed to thermal transport and that thermal contacts between CNTs within the array had a negligible effect. Huxtable et al. [33] found G ~12 MW m −2 K −1 for individual surfactant-coated single-wall CNTs dispersed in water. For graphene, which is more amenable to direct measurement of G than CNT-based materials because of its planar geometry, Schmidt et al. [34] was able to use TDTR to measure interface conductance between several metals and HOPG, obtaining room-temperature values from 30 to 100 MW m −2 K −1 for the basal plane. By the same technique, Koh et al. [35] obtained 25 MW m −2 K −1 between Au/Ti and few-layer graphene. Chen et al. [36] used the 3-omega method to investigate the graphene–silicon oxide interface, obtaining 18–83 MW m −2 K −1 . Tong et al. [28] obtained an effective resistance of 10 mm 2 K W −1 for a CNT array pressed against a non-functionalized substrate. These values are consistent with our measured G for non-functionalized CNT arrays of 50–80 W m −2 K −1 but are difficult to compare directly to our study since we do not know whether the array CNT contacts are predominately end-on or side contacts with short CNT segments parallel to the interface. Cola et al. [37] have discussed mechanical models for the latter type of contacts within CNT arrays. We do not make any specific assumptions about the precise contact geometry. Our analysis determines an intrinsic value for the CNT interface conductance G proportional to σ contact , the effective heat capacity relative to that of HOPG, or in other words proportional to the cross-sectional area of the CNTs contributing to thermal transport. Although our approach has substantially improved the interface G through the control of interface chemistry, σ contact remains relatively small because of the inhomogeneities of the length and orientation of individual CNTs within CVD-grown arrays. If a means can be found to make contact to a majority of CNTs within an array, there is room for a further order of magnitude reduction in the effective array thermal interface resistance. The chemical nature of heteromaterial interfaces has a decisive effect on thermal transport in nanoscale systems. We have shown that bridging the CNT–metal interface with covalent linkers substantially increased both thermal transport and mechanical interface adhesion relative to that resulting from the van der Waals interactions between unmodified CNTs and metals. This confirms Prasher’s model [15] for thermal transport at van der Waals contacts and the molecular dynamics results of Hu et al. [38] Losego et al. [39] recently showed that the thermal interface resistance between a gold film and a self-assembled monolayer (SAM) on quartz could be halved by changing the SAM head-group from methyl to thiol. Our functionalization scheme for aligned CNT arrays is robust, stable against aging and thermal stress, and adaptable to both noble and more reactive metals. This development may lead to the practical application of aligned CNT arrays for thermal management in microelectronic devices. CNT growth MWCNT arrays were grown on Si substrates by CVD using both a 5-cm tube furnace and an automated wafer-scale CVD system for carbon-based material growth (Aixtron Black Magic Pro). A detailed description of the process can be found elsewhere [40] . Briefly, a 10-nm thick Al 2 O 3 layer and a 2-nm thick Fe layer were deposited on the Si wafer by e-beam evaporation. MWCNT arrays were grown in the tube furnace at 770 °C using ethylene as the carbon source or in the Aixtron system at 680 °C using acetylene. Electron microscope images of MWCNT arrays are shown in Supplementary Fig. 1 . CNT diameters were 18 nm and lengths were 70–100 μm. Functionalization and bonding After CVD growth, MWCNT arrays were oxidized in air plasma (Harrick Plasma, Model PDC-32G) at 50 mTorr for 5 min. Plasma treatment helped to remove the amorphous carbon over-layer, which is usually present at the surface of CVD-grown arrays, and also oxidized the surface region for subsequent functionalization [41] . XPS spectra are shown in Supplementary Fig. 2 . For functionalization, glass microscope cover slips were coated with either a 5-nm Ti adhesion layer followed by 70 nm of Al or by 140 nm of Au using e-beam evaporation then cleaned for 20 min in a 200-mTorr O 2 plasma prior to functionalization. Pure oxygen was used since cleaning in air plasma resulted in fluorine passivation of the Al surface by trace fluorocarbons in the ambient air. To functionalize with APS, Al coupons were dipped into a 0.1 V/V solution of APS in ethanol for 5 min followed by an ethanol rinse. APS was purchased from Sigma-Aldrich and used as received. Al-coated Si substrates were functionalized in a similar way for adhesion testing. For cysteamine functionalization, Au coupons were dipped into a 1-mM toluenic solution of cysteamine for 15 min followed by toluene rinse. Cysteamine and toluene were purchased from Sigma-Aldrich and used as received. Gold-covered Si substrates were functionalized in a similar way for adhesion testing. Surface functionalization was confirmed using XPS ( Supplementary Fig. 3 ). After functionalization, substrates were dried under vacuum for 20 min at 120 °C, then placed against plasma-treated MWCNT arrays, clamped together at ~0.5 bar, and then heated to 120 °C for 1 h. Non-functionalized control samples were prepared under similar conditions by pressing plasma-cleaned Al or Au films to as-grown (control 1) or plasma-treated (control 2) MWCNT arrays. Adhesion testing MWCNT array–metal interface adhesion was measured using a lab-built apparatus consisting of a 500-g load cell (Transducer Techniques GS0-500) and a stepper-motor-driven micrometre with sub-micrometre resolution (Newport NewStep NSC200). Tensile loads were applied perpendicular to the MWCNT interface. A linear stress–strain response was observed, corresponding to the compliance of the load cell, until the interface failed. Yield stress was calculated from the applied tensile load and MWCNT contact area, determined after failure from scanning electron microscope images. Yield stress for functionalized samples (both APS-Al and cysteamine-Au) ranged from 43 to 70 kPa, and failure occurred at the CNT growth interface, resulting in a complete transfer of the aligned MWCNT arrays from the growth substrates to functionalized contact substrates. Most non-functionalized control assemblies failed spontaneously under their own weight when the clamping load was removed after bonding, indicating interface strength below 0.1 kPa. Some control samples sustained stresses up to ~8 kPa, with failure occurring at the contact interface instead of the growth substrate. Experimental data from adhesion testing are shown in Supplementary Fig. 4 . The complete MWCNT array transfer from the growth to the functionalized surface after adhesion testing is shown in Supplementary Fig. 5 . Thermal characterization We used a modified version of the TDTR [13] method to characterize interfacial thermal transport. A 76-MHz train of fs (pump) pulses at 830 nm from a Ti-sapphire laser heated the metal film by a few degrees, and the same laser drove an optical parametric oscillator producing a synchronized, variable wavelength (probe) pulse train used to measure the film temperature. Coaxial pump and probe beams with independently adjustable diameters were focused on the same via a × 20 objective. Spot sizes and alignments were imaged through the same objective. The pump laser was modulated at 0.8, 2.3 or 9 MHz with an electro-optic modulator. The phase and amplitude of the probe response at the pump modulation frequency were measured as functions of pump–probe delay with a fast photodiode detector, filtered to reject scattered pump light and connected through a resonant RLC filter to a 400-MHz preamplifier and a radio-frequency lock-in amplifier. The lock-in phase was adjusted so the jump in thermal response at delay time zero occurred only in the in-phase channel. The probe laser was operated at 725 nm for Al films or 555 nm for Au films to optimize the thermo-reflectance sensitivity. The phase-shift depends on experimental parameters (pump modulation frequency and laser spot diameters) and the thermal properties of the multilayered sample (thickness, thermal conductance, heat capacity and interface resistance for each layer) [20] . The pump spot diameter was set to 28 μm and the probe spot was ~4 μm. Thermal modelling Experimental TDTR data were compared with model calculations based on the multilayer radial-symmetry heat flow model of Cahill [20] combined with the bidirectional heat-flow analysis of Schmidt et al. [21] The pump spot diameter, metal–glass interface conductance and glass thermal conductivity were determined by multifrequency fits to TDTR measurements on the metal substrates alone as shown in Supplementary Fig. 6 . Difference in TDTR data inside and outside the CNT contacts are then only because of the CNT–metal interface resistance and the thermal properties of the CNT array. Literature values were used for the bulk thermal properties of Al and Au films and vendor specifications for the glass heat capacity. The metal film thickness was independently determined from pico-acoustic echos [42] . The Al metal–glass interface conductance of 175 MW m −2 K −1 and the pump beam diameter of 28 μm (consistent with independent optical measurements) were determined by fitting the multifrequency reference data. Identical fitting parameters were then used for the metal–glass thermal properties for both signal and reference data. Under our conditions, the length of the CNT array can be considered semi-infinite as the MHz thermal waves do not penetrate to the Si growth substrate. The CNT array was parameterized by its mass density (contact percentage) relative to HOPG. Dense, vertically aligned CNT arrays typically have 10% of HOPG density; however, only a fraction of the CNT array was assumed to contribute to thermal transport. MWCNT heat capacity was assumed to be equal to HOPG, 1.91 MJ m −3 K −1 (ref 34 ), adjusted for contact percentage. Axial MWCNT conductivity was assumed to be 2,000 W m −1 K −1 , with the effective CNT array conductivity adjusted for contact percentage. Lateral CNT array conductivity was set to zero, although this had a negligible effect on calculated phase shifts. The interface G was also adjusted for contact percentage. G therefore represents an intrinsic property of the CNT array. For example, if 5% of the CNT in a 10% dense array contributed to thermal transport, the CNT layer-effective heat capacity is 0.005 that of HOPG, its Λ is 0.005 of 2,000 W m −1 K −1 , and its effective G is 0.005 of the intrinsic G . Repeating the model calculations with a CNT axial conductivity of 3,000 W m −1 K −1 gave almost the same results as for 2,000 W m −1 K −1 , with a slight reduction in the CNT contact fraction. In many cases, a least-squares minimization procedure is used to adjust model parameters to fit experimental TDTR data. This only works if there are independent responses to variations in different parameters leading to a unique minimum in parameter space. This fails for our experiment since [ G , σ ] are coupled for single-frequency differential TDTR of the CNT array contacts. We resolve this problem through multifrequency TDTR experiments [43] , which now lead to a unique solution for G and σ , as shown in Supplementary Fig. 7 . How to cite this article: Kaur, S. et al. Enhanced thermal transport at covalently functionalized carbon nanotube array interfaces. Nat. Commun. 5:3082 doi: 10.1038/ncomms4082 (2014).